A multitasking functional group leads to structural diversity using designer C–H activation reaction cascades The C–H activation strategy has become one of the preferred methods to introduce chemical functionality to a chemically inert carbon atom. Intensive efforts have been devoted to developing either versatile bond formations (product structural diversity) or effective directing groups (substrate site selectivity). From the views of medicinal and synthetic practitioners, the C–H activation approach remains inadequate due to its limitation to point-to-point derivatization. Direct assembly of 3D molecular complexity in a single step remains elusive for this strategy. Towards this goal, a multitasking functional group is required to accomplish several missions in one pot: site selecitivity, cleavability and redox versatility. We demonstrate that an oxyacetamide group is such a multifunctional warhead that enables a series of C–H functionalization cascades and allows direct access to structurally diverse polycyclic heterocyles in one pot. The progress of these reaction cascades were fully controlled by oxidants and temperature. The proliferation of the reaction chain can be extended to a four-step cascade. C–H activation reactions refer to a carbon–hydrogen bond cleavage process mediated by organometallics, where the bond dissociation is accomplished through coordination of the C–H bond to the inner sphere of a transition metal [1] , [2] , [3] . In this paradigm, directed C–H functionalization received the most attention, as a coordinative group (directing group, DG) on a substrate can escort the transition metal in proximity to one specific C–H bond, resulting in precise site-selective control among many innocent hydrocarbons [4] , [5] , [6] . However, the use of a DG often leaves a chemical trace in the products, limiting their structural diversity ( Fig. 1a ). [7] Strategies trying to address this drawback include incorporation of the DG into a heterocycle via in situ condensation reactions or development of a traceless DG [8] , [9] , [10] , [11] , [12] , [13] , [14] , [15] , [16] . For example, we have developed a fully cleavable DG that allowed both convenient removal and conversion to various functional groups after the C–H activation step. The triazene group was discovered as an excellent DG for ortho C–H rhodation and subsequent chemical manipulations. This group can be removed quantitatively or undergo a number of C–C, C–O, C–N and C–X bond formation, leaving no trace in the products ( Fig. 1b ). [8] In addition, the triazene could also engage in heterocyclization with internal alkynes via partial in situ cleavage to generate substituted indole analogues [9] . Recently, Ellman, Bergman and colleagues [10] described a rhodium-catalysed annulation reaction between an azobenzene and an azidobenzene to yield a substituted phenazine. A Friedel–Crafts type of in situ electrophilic cyclization/aromatization sequence was used to incorporate the DG into the heterocycle ( Fig. 1c ). Despite these advances, the structural diversity of the C–H functionalization products remains convergent. In addition, the chemistry involving DGs post the pivotal C–H activation reaction remains underexplored. Therefore, a strategy allowing for rapid construction of 3D molecular architecture using the C–H activation concept would require a multipurpose functional group: first, it can serve as an excellent binder for transition metals and dictates site selectivity; second, it is labile and readily cleavable; third, it is redox versatile and enables inter- and intramolecular ring formation. 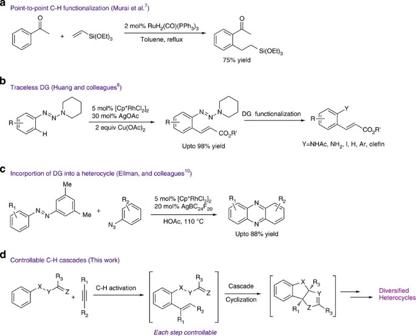Figure 1: Evolution of the C–H activation strategy. (a) The first catalytic C–H activation reaction was developed by Muraiet al.7(b) The traceless triazene DG developed by us8,9. (c) A representative example of DG incorporates into a heterocycle: phenazine synthesis by Ellman, Bergman and colleagues10. (d) Our multitasking strategy to access highly sophisticated heterocyclic scaffold containing two quaternary stereogenic centers that might allow further ring formations. Figure 1: Evolution of the C–H activation strategy. ( a ) The first catalytic C–H activation reaction was developed by Murai et al. [7] ( b ) The traceless triazene DG developed by us [8] , [9] . ( c ) A representative example of DG incorporates into a heterocycle: phenazine synthesis by Ellman, Bergman and colleagues [10] . ( d ) Our multitasking strategy to access highly sophisticated heterocyclic scaffold containing two quaternary stereogenic centers that might allow further ring formations. Full size image Ideally, the multifunctional DG participates in a number of reaction cascades in the presence of an orthogonal catalyst/additive, and therefore substantially enriches the molecular complexity of the products. Preferably, the reaction cascades can be controlled by either the catalyst or additives, rendering designated proliferation of the reaction chain. Towards this goal, we envisioned that the O-NHAc (oxyacetamide) fulfills the multifunctional criteria of such a group due to its excellent metal directing ability, the oxidative O–N bonds and nucleophilic amide functionality [11] , [12] , [13] , [14] . We chose the rhodium catalysed C–H vinylation reaction between an N -aryloxyacetamide and an internal alkyne to explore the cascade strategy [17] , [18] , [19] . After the C–H vinylation, the oxyacetamide DG might undergo transition-metal-catalysed dioxygenation reaction to give rise to a fused dihydrofuran–dihydrooxazole scaffold. This [5,5] heterocycle contains a chemically labile hemiaminal functionality and is likely to trigger several rearrangement/oxidation pathways to give substituted polyheterocycles. Therefore, such a multitasking functional group of will open doors to rapid structural diversification through multistep cascades using simple substrates. The double cascade towards dihydrobenzofuro[2,3– d ]oxazoles We embarked on our design by investigating a reaction between N -phenoxyacetamide ( 1a ) and diphenylacetylene ( 2a ), which was recently published by Lu and co-workers to undergo a classic point-to-point ortho-selective vinylation reaction and yield the enamide product ( 3aa ) [11] . Treatment of 3aa with various transition metals in an attempt to cyclize the oxyacetamide onto the double bond quickly identified that using 1.2 equiv. Ag 2 CO 3 alone, a new heterocycle was formed in quantitative yield. Single crystal X-ray crystallography confirmed an unusual dioxygenation of the olefin, leading to a dihydrobenzofuro[2,3– d ]oxazole skeleton bearing two adjacent quaternary stereogenic centres as a single diastereomer. The mechanism of this transformation is intriguing as 1 equiv. of H 2 was observed. Presumably, a phenoxylation catalysed by silver is followed by a rapid dehydrogenative cyclization [20] , [21] , [22] , [23] . Detailed mechanistic aspects are currently under investigation ( Fig. 2 ). 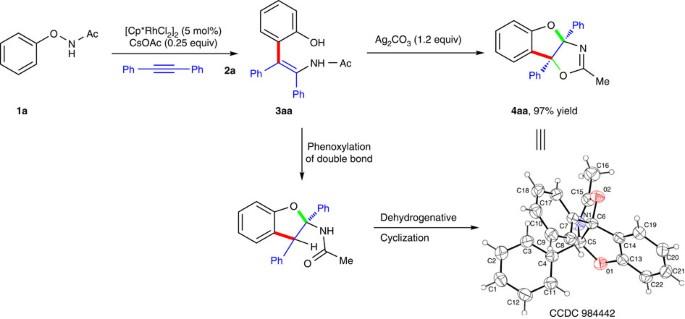Figure 2: Oxidative cyclization of enamide3aa. Unusual silver promoted oxidative cyclization of enamide3aa. Figure 2: Oxidative cyclization of enamide 3aa . Unusual silver promoted oxidative cyclization of enamide 3aa . Full size image Scope of arenes for the double cascade Encouraged by the formation of 4aa , we attempted to combine this dioxygenative cyclization with the initial C–H vinylation condition in a one pot cascade. Gratifyingly, 5 mol% [RhCp*Cl 2 ] 2 and 1.2 equiv. of Ag 2 CO 3 in MeOH at 25 °C smoothly converted N -phenoxyacetamide ( 1a ) to the desired dihydrobenzofuro[2,3– d ]oxazole 4aa directly in 97% isolated yield. To the best of our knowledge, this is the first example of the heterocycle containing two chiral centres prepared in one pot via a C–H activation process. The reaction did not proceed in the absence of Rh. The substrate scope was examined next. A series of substituted aryloxyacetamides smoothly reacted with diphenylacetylene 2a to afford the desired heterocyles ( Table 1 ). Yields of those bearing electron-donating substituents were particularly high. The reaction of a substrate having an electron-withdrawing CF 3 was sluggish (41% yield). The dimethyl-substituted substrate 1f resulted in moderate yield (68%). Halogens, including iodine, were well tolerated and the corresponding halogenated dihydrobenzofuro[2,3– d ]oxazoles were isolated in yields ranging from 75 to 79%. Single regioisomeric product was obtained when a meta-substituted N -phenoxyacetamide was used. The oxyacetamide DG allowed bulky substituent and yield was uncomprised. Table 1 Substrate scope of aryloxyacetamide for one-pot synthesis of dihydrobenzofuro[2,3– d ]oxazoles. Full size table Scope of alkynes for the double cascade The scope of alkynes was also surveyed ( Table 2 ). A series of aryl-substituted alkynes coupled with 1a smoothly and the relevant products were isolated in moderate yield (60–75%). Unsymmetrical internal alkynes were also effective, generating single regioisomeric products. X-ray crystallography analysis (for 4ad , see Supplementary Information ) revealed that the alkyl group is pointed distal to the nitrogen atom. Dialkyl-substituted alkynes failed to react with 1a under standard condition. On the other hand, electron-deficient internal alkynes, 3-phenylpropiolonitrile for example, reacted smoothly and the desired dihydrobenzofuro[2,3– d ]oxazole was obtained in 40% yield. Table 2 Substrate scope of alkynes for one-pot synthesis of dihydrobenzofuro[2,3– d ]oxazoles. Full size table The double cascade towards polysubstituted isoquinoline Next, we attempted to further increase the molecular complexity by treating the dihydrobenzofuro[2,3– d ]oxazole product 4 with another alkyne under C–H activation conditions. Interestingly, a polysubstituted isoquinoline product 5 was obtained, through a C–H annulation/rearrangement process. The formation of 5 from 4 required the employment of AgTFA (2.2 equiv.) and methanol at 120 °C. Both aryl,aryl- and alkyl,alkyl-disubstituted alkynes were tolerated and the products were obtained in moderated yields. Separate experiments show that the formation of 5 probably goes through intermediate 3 , as 4 was converted back to 3 at 120 °C in the absence of alkyne ( vide infra ). 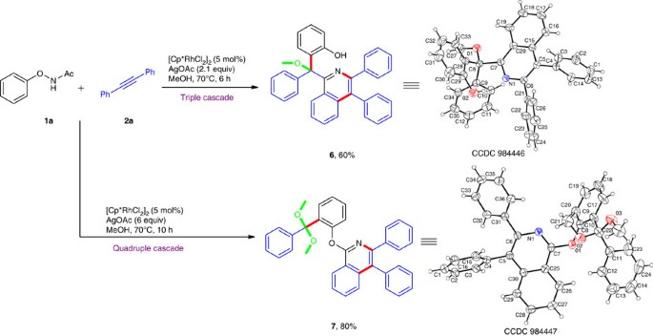Figure 3: Multistep cascade reactions. Conditions for6:N-phenoxyamide (0.2 mmol), diphenylacetyene (0.44 mmol), [RhCp*Cl2]2(5 mol%), AgOAc (2.1 equiv.), MeOH (1 ml), isolated yield. Conditions for7:N-phenoxyamide (0.2 mmol), diphenylacetyene (0.44 mmol), [RhCp*Cl2]2(5 mol%), AgOAc (6 equiv.), MeOH (1 ml), isolated yield. Based on this finding, conditions were tested to access the dihydrobenzofuro[2,3– d ]oxazole product 5 directly from N -phenoxyacetamide 1 and excess alkyne 2 ( Table 3 ). We were delighted to find that the reaction proceeded smoothly using [Cp*RhCl 2 ] 2 (5 mol%), AgTFA (2.2 equiv.) and CsOAc (2 equiv.) at 120 °C. Interestingly, the overall yield for the 1 – 5 triple cascade was generally higher than that of the single-step reaction of 4–5 . Unsymmetrical internal acetylenes led to single regioisomers, whose configuration was determined by X-ray. This double cascade demonstrated substantial increase of structural complexity for a one-pot reaction using very simple starting materials. Table 3 Substrate scope of polysubstituted isoquinoline product 5. Full size table The double cascade using two different alkynes in one pot A major limitation for the one-pot cascade in Table 3 is that the same alkyne reacts twice, which restricts the structure diversification of the product. However, subjecting two different alkynes to the reaction condition ( Table 3 ) resulted in messay mixtures. After a quick condition survey, we were excited to find that sequential addition of alkynes provided a nice solution to the chemoselectivity issue. First, N -phenoxyacetamide 1 was mixed with 1.05 equiv. 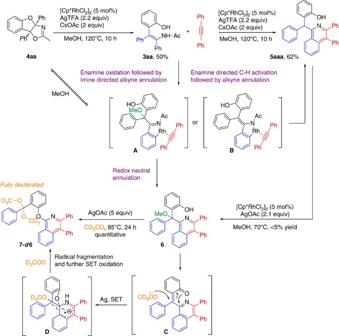Figure 4: Mechanistic studies and proposed mechanisms for the formation of5,6and7. The formation of5aaafrom4aais believed to occur via intermediate3aa. Product6cannot be obtained by direct oxidation of5aaa, probably due toin situoxidation of the intermediates. We propose a radical fragmentation mechanism for the formation of7from6. SET, single-electron transfer. alkyne A at room temperature; next, the second alkyne B was introduced on consumption of A and the reaction temperature was raised 120 °C ( Table 4 ). This experimental maneuvre led to clean isolation of the hybrid product. No other isomers were observed. Interestingly, the other double-cascade product 4 was not observed throughout the course of the cascade, suggesting that the formation of 5 did not necessarily go through 4 as a key intermediate. Table 4 Double cascade using two different alkynes. Full size table Triple and quadruple cascades As the isoquinoline product 5 contains a redox-labile triaryl methine moiety, we examined the feasibility of obtaining further functionalized product of higher oxidation states directly from 1a . Gratifyingly, treating N -acetyl phenyloxyamide 1a and excess diphenyl acetylene with [Cp*RhCl 2 ] 2 , AgOAc (2.1 equiv.) in methanol led to the corresponding methyl ether product smoothly, rendering a three-step (C–H vinylation, C–H annulation and oxidation) cascade reaction. Simply increasing the amount of oxidant to 6 equiv. afforded the corresponding dimethyl ketal product in 80% yield, a quadruple cascade. The termination of these cascades was precisely controlled by the silver oxidant and its stoichiometry. The mechanisms for the formation of 5 , 6 and 7 are intriguing. A series of experiments were carried out to further understand these transformations. Treatment of 4aa with the Rh catalyst, AgTFA and CsOAc at 120 °C led to the formation of enamide 3aa in 50% isolated yield. Treating 3aa with [Cp*RhCl 2 ] 2 and AgOAc, in the absence of the alkyne, generated 4aa in high yield at 70 °C, which went back to 3aa and its double-bond isomer ( trans -enamide) when further heated at 120 °C. The enamide product 3aa readily reacted with diphenyl acetylene to yield dihydrobenzofuro[2,3– d ]oxazole 5aaa in 62% yield. This result suggests that the formation of 5aaa from 4aa is likely to occurr via intermediate 3aa . The absence of 4 for the one-pot reaction using two different alkynes ( Table 4 ) also supports that 4 is not involved for in the cascade from 1 to 5 . Careful examination of the cascade mixture led to the detection of 3 that slowly converted to 5 on addition of the second alkyne. The mechanism for 3aa to 5aaa probably involves C–H activation using NHAc as the DG (Fig. 4, intermediate B ), which is well documented for reactions with internal alkynes [24] , [25] . Treatment of 5aaa under various oxidative conditions afforded very little 6 , suggesting that direct oxidation of 5aaa is not responsible for the formation of 6 . This is also supported by the fact that the direct formation of 6 from 1a requires lower temperature than 5aaa from 1 . A more plausible explanation for the triple cascade product 6 ( Fig. 3 ) is the in situ enamine oxidation of the 3aa to its corresponding α-methoxy imine (possibly in equilibrium with 4aa ), which directs the subsequent C–H annulation reaction with the alkyne ( Fig. 4 , intermediate A ). Treatment of 6 with CD 3 OD and excess AgOAc (5 equiv) yielded fully deuterated dimethyl ketal 7- d 6 . We propose a silver mediated single-electron transfer (SET) process for this rather unusual oxidative rearrangement. On phenolate addition to the pyridine ring, the resulting dihydropyridine C could be readily oxidized by silver to generate a conjugated radical cation D . This radical cation could undergo β-fragmentation to yield a more stable α-methxoy diarylmethyl radical. Further oxidation of this radical, followed by CD 3 OD addition would afford the desired 7- d 6 . This unprecedented carbon–carbon cleavage is under investigation using simple substrates to test its synthetic generality. Figure 3: Multistep cascade reactions. Conditions for 6 : N -phenoxyamide (0.2 mmol), diphenylacetyene (0.44 mmol), [RhCp*Cl 2 ] 2 (5 mol%), AgOAc (2.1 equiv. ), MeOH (1 ml), isolated yield. Conditions for 7 : N -phenoxyamide (0.2 mmol), diphenylacetyene (0.44 mmol), [RhCp*Cl 2 ] 2 (5 mol%), AgOAc (6 equiv. ), MeOH (1 ml), isolated yield. Full size image Figure 4: Mechanistic studies and proposed mechanisms for the formation of 5 , 6 and 7 . The formation of 5aaa from 4aa is believed to occur via intermediate 3aa . Product 6 cannot be obtained by direct oxidation of 5aaa , probably due to in situ oxidation of the intermediates. We propose a radical fragmentation mechanism for the formation of 7 from 6 . SET, single-electron transfer. Full size image In summary, we develop a series of C–H functionalization cascades catalysed by Rh(III), which enable direct access to several heterocyclic scaffolds using oxyacetamide as a multitasking group. This enzyme-like rapid proliferation of reaction cascades, up to four steps, features unprecedented dioxygenation, oxidation and rearrangement mechanisms that are fully controlled by the choice of silver oxidant, its equivalence and reaction temperature. The reactions show excellent chemoselectivity and wide substrate scope for both N -aryloxyamides and internal alkynes. The products showed substantially increased molecular complexity and steady elevation of oxidation state. We expect that this strategy will offer endless opportunities for rapid assembly of structurally diverse heterocycles using the C–H activation strategy. Materials All reagents were purchased and used without further purification unless otherwise specified. Solvents for flash column chromatography were technical grade and distilled before use. Analytical thin-layer chromatography was performed using silica gel plates with HSGF 254 (0.15–0.2 mm) manufactured by Shandong Huanghai Chemical Company (Qingdao, China). Visualization of the developed chromatogram was performed by measuring ultraviolet absorbance (254 nm) and using appropriate stains. Flash column chromatography was performed using Qingdao Haiyang Chemical HG/T2354-92 silica gel (45–75 μm) with the indicated solvent system according to standard techniques. General spectroscopic methods 1 H NMR and 13 C NMR data were recorded on Bruker 400 MHz (100 MHz for 13 C) nuclear resonance spectrometers unless otherwise specified. Chemical shifts ( δ ) in p.p.m. are reported relative to the residual signals of chloroform ( 1 H 7.26 p.p.m. and 13 C 77.16 p.p.m.). Multiplicities are described as follows: s (singlet), bs (broad singlet), d (doublet), t (triplet), q (quartet) and m (multiplet). Coupling constants ( J ) are reported in Hertz (Hz). 13 C NMR spectra were recorded with total proton decoupling. High-resolutionmass spectrometry–electrospray ionization (HRMS–ESI) analysis was performed by the Analytical Instrumentation Center at Peking University, and HRMS data were reported as ion mass/charge (m/z ) ratios in atomic mass units. 1 H NMR, 13 C NMR and HRMS are provided for all compounds; see Supplementary Figs 1–79 . For oak ridge thermal ellipsoid plot (ORTEP) presentation of 4aa , 4ad , 5aaa , 5aak , 6 and 7 , see Supplementary Figs 79–85 . See Supplementary Methods for the characterization data for compounds not listed in this section. See Supplementary data 1–6 for X-ray CIF files of compounds 4aa , 4ad , 5aaa , 5aak , 6 and 7 (CCDC 984442-984447). One-pot synthesis of 4aa Without precaution to extrude air or moisture, N -phenoxyacetamide 1a (0.5 mmol, 1 equiv. ), diphenyl acetylene (0.6 mmol, 1.2 equiv. ), [Cp*RhCl 2 ] 2 (0.025 mmol, 5 mol%) and Ag 2 CO 3 (1.2 equiv.) were weighted in a 1-dram vial equipped with a stir bar. MeOH (1.25 ml) was added. The reaction was stirred at room temperature for 12 h, diluted with dichloromethane and transferred to a round-bottom flask. Silica gel (0.5 g) was added to the flask and the reaction vessel was concentrated under reduced pressure. The silica gel-absorbed product was purified by silica gel flash column chromatography to yield 4aa (97% yield). 1 H NMR (300 MHz, CD 2 Cl 2 ): δ 7.51–7.42 ( m , 1H), 7.23–7.03 ( m , 11H), 6.98–6.87 ( m , 2H), 2.32 ( s , 3H); 13 C NMR (75 MHz, CD 2 Cl 2 ): δ 169.48, 159.69, 137.57, 137.10, 131.74, 127.91, 127.59, 127.52, 127.37, 126.95, 126.89, 126.42, 121.99, 117.49, 110.88, 99.15, 14.37; HRMS (ESI) calculated for [C 22 H 18 NO 2 ] + : 328.1338; Found: 328.1331; infrared (cm −1 ): 3061.00, 1662.64, 1598.99, 1463.97, 1282.66, 1001.06, 752.24, 696.30. One-pot synthesis of 5aaa N -phenoxyacetamide 1a (0.5 mmol, 1 equiv. ), diphenyl acetylene (0.6 mmol, 1.2 equiv. ), [Cp*RhCl 2 ] 2 (0.025 mmol, 5 mol%), AgTFA(1.1 mmol, 2.2 equiv. ), CsOAc (1 mmol, 2 equiv.) and MeOH (1.25 ml) were added to a sealed tube in a glovebox. The reaction was stirred at 120 °C for 8 h, before it was diluted with dichloromethane and transferred to a round-bottom flask. Silica gel (0.5 g) was added to the flask and the reaction vessel was concentrated under reduced pressure. The silica gel absorbed product was purified by silica gel flash column chromatography to yield 5aaa (73% yield). 1 H NMR (300 MHz, CD 2 Cl 2 ): δ 12.10 ( s , 1H), 8.72–8.56 ( m , 1H), 8.72–8.56 ( m , 1H), 7.84–7.72 ( m , 3H), 7.53 ( d , J =7.0 Hz, 1H), 7.43 ( s , 3H), 7.29 (dt, J =17.5, 7.5 Hz, 11H), 7.16 (d, J =7.0 Hz, 2H), 7.01–6.88 ( m , 2H), 6.56 ( s , 1H); 13 C NMR (75 MHz, CD 2 Cl 2 ): δ 161.86, 157.19, 141.75, 139.21, 137.37, 136.65, 132.16, 131.49, 131.24, 131.05, 130.15, 129.42, 128.43, 128.30, 128.18, 128.00, 127.87, 127.82, 127.76, 127.70, 127.61, 126.87, 126.47, 125.92, 124.70, 119.56; HRMS (ESI) calculated for [C 34 H 26 NO] + : 464.2014; Found: 464.2000. infrared (cm −1 ): 3057.17, 2358.94, 1556.55, 1487.12, 1379.10, 1255.66, 759.95, 732.95, 698.23. One-pot synthesis of 5aak N -phenoxyacetamide 1a (0.5 mmol, 1 equiv. ), diphenyl acetylene (0.6 mmol, 1.2 equiv. ), [Cp*RhCl 2 ] 2 (0.025 mmol, 5 mol%), AgTFA(1.1 mmol, 2.2 equiv.) and Ag 2 CO 3 (1.2 equiv.) were weighted in a 1-dram vial equipped with a stir bar. MeOH (1.25 ml) was added. The reaction was stirred at room temperature for 12 h. Next, 3-hexyne (1.0 mmol, 2.0equiv) was added. The reaction was stirred at 120 °C for 8 h, before it was diluted with dichloromethane and transferred to a round-bottom flask. Silica gel (0.5 g) was added to the flask and the reaction vessel was concentrated under reduced pressure. The silica gel absorbed product was purified by silica gel flash column chromatography to yield 5aak (48% yield). 1 H NMR (400 MHz, CD 2 Cl 2 ): δ 12.88 ( s , 1H), 8.50 ( d , J =8.5 Hz, 1H), 8.16 ( d , J =8.6 Hz, 1H), 7.82 ( t , J =7.6 Hz, 1H), 7.67 ( t , J =7.6 Hz, 1H), 7.50–7.41 ( m , 1H), 7.28–7.17 ( m , 4H), 7.02 (d, J =7.0 Hz, 2H), 6.96 ( d , J =7.8 Hz, 1H), 6.89 ( t , J =7.4 Hz, 1H), 6.36 (s, 1H), 3.14 (dd, J =7.6, 2.1 Hz, 2H), 3.09–2.96 (m, 2H), 1.34 (td, J =7.5, 2.4 Hz, 6H); 13 C NMR (101 MHz, CD 2 Cl 2 ): δ 159.88, 157.39, 151.26, 142.12, 136.42, 132.10, 130.75, 129.76, 129.24, 128.28, 128.01, 127.75, 126.75, 126.25, 125.71, 125.21, 124.03, 119.51, 119.27, 27.62, 20.72, 14.87, 14.38; HRMS (ESI) calculated for [C 26 H 26 NO] + : 368.2014; Found: 368.2010. One-pot synthesis of 6 N -phenoxyacetamide 1a (0.5 mmol, 1 equiv. ), diphenyl acetylene (0.6 mmol, 1.2 equiv. ), [Cp*RhCl 2 ] 2 (0.025 mmol, 5 mol%), AgOAc (1.05 mmol, 2.1 equiv.) and MeOH (1.25 ml) were added to a a sealed tube in a glovebox. The reaction was stirred at 70 °C for 6 h, before it was diluted with dichloromethane, and transferred to a round-bottom flask. Silica gel (0.5 g) was added to the flask and the reaction vessel was concentrated under reduced pressure. The silica gel absorbed product was purified by silica gel flash column chromatography to yield 6 (60% yield). 1 H NMR (400 MHz, CD 2 Cl 2 ): δ 9.82 ( s , 1H), 9.14 ( d , J =7.5 Hz, 1H), 7.77 ( d , J =7.7 Hz, 1H), 7.75–7.71 ( m , 1H), 7.64–7.54 ( m , 2H), 7.47–7.43 ( m , 3H), 7.43–7.37 ( m , 6H), 7.31 (d, J =1.5 Hz, 1H), 7.30–7.28 (m, 1H), 7.25 (d, J =4.9 Hz, 1H), 7.19 (dd, J =10.7, 4.4 Hz, 4H), 6.98–6.91 (m, 1H), 6.80 ( d , J =7.7 Hz, 1H), 3.18 ( s , 3H); 13 C NMR (101 MHz, CD 2 Cl 2 ): δ 158.42, 155.34, 146.40, 140.49, 139.56, 138.15, 137.04, 131.72, 131.48, 130.90, 130.26, 130.14, 129.70, 129.32, 128.54, 128.25, 127.72, 127.67, 127.62, 127.47, 127.39, 127.20, 126.84, 126.55, 125.51, 119.33, 118.72, 90.97, 29.71; HRMS (ESI) calculated for [C 35 H 28 NO 2 ] + : 494.2120; Found: 494.2117; infrared (cm −1 ): 3055.24, 2358.94, 1577.77, 1446.61, 1242.16, 1074.35, 763.81, 700.61, 669.30. One-pot synthesis of 7 N -phenoxyacetamide 1a (0.5 mmol, 1 equiv. ), diphenyl acetylene (0.6 mmol, 1.2 equiv. ), [Cp*RhCl 2 ] 2 (0.025 mmol, 5 mol%), AgOAc (1.05 mmol, 2.1 equiv.) and MeOH (1.25 ml) were added to a a sealed tube in a glovebox. The reaction was stirred at 70 °C for 6 h, before it was diluted with dichloromethane, and transferred to a round-bottom flask. Silica gel (0.5 g) was added to the flask and the reaction vessel was concentrated under reduced pressure. The silica gel absorbed product was purified by silica gel flash column chromatography to yield 7 (80% yield). 1 H NMR (400 MHz, CD 2 Cl 2 ): δ 8.18 (dd, J =7.8, 1.7 Hz, 1H), 8.00 ( d , J =7.8 Hz, 1H), 7.67–7.61 ( m , 1H), 7.60–7.51 ( m , 2H), 7.45–7.41 ( m , 1H), 7.40–7.33 ( m , 6H), 7.23 (ddd, J =7.8, 5.0, 1.5 Hz, 3H), 7.17–7.13 ( m , 1H), 7.13–7.06 ( m , 7H), 3.06 (s, 6H); 13 C NMR (101 MHz, CD 2 Cl 2 ): δ 158.61, 150.58, 146.47, 141.36, 140.51, 138.70, 137.92, 134.38, 131.53, 130.54, 130.11, 129.12, 128.96, 128.27, 127.49, 127.16, 127.13, 127.04, 126.73, 126.14, 125.80, 125.17, 124.63, 124.61, 124.32, 118.18, 101.02, 48.92; HRMS (ESI) calculated for [C 35 H 27 NO 2 Na] + : 546.2045; Found: 546.2037. infrared (cm −1 ): 3059.10, 2937.59, 2358.94, 1620.21, 1573.91, 1373.32, 1213.23, 1056.99, 767.67, 700.16. Accession codes: The X-ray crystallographic coordinates for structures reported in this study have been deposited at the Cambridge Crystallographic Data Centre (CCDC), under deposition numbers CCDC 984442–984447. These data can be obtained free of charge from The Cambridge Crystallographic Data Centre via www.ccdc.cam.ac.uk/data_request/cif . How to cite this article: Chen, Y. et al. A multitasking functional group leads to structural diversity using designer C–H activation reaction cascades. Nat. Commun. 5:4610 doi: 10.1038/ncomms5610 (2014).